Diastereoselective desymmetric 1,2-cis-glycosylation ofmeso-diols via chirality transfer from a glycosyl donor Chemical desymmetrization reactions of meso -diols are highly effective for the precise and efficient synthesis of chiral molecules. However, even though enzyme-catalyzed desymmetric glycosylations are frequently found in nature, there is no method for highly diastereoselective desymmetric chemical glycosylation of meso -diols. Herein, we report a highly diastereoselective desymmetric 1,2- cis -glycosylation of meso -diols found in myo -inositol 1,3,5-orthoesters using a boronic acid catalyst based on predictions of regioselectivity by density functional theory (DFT) calculations. The enantiotopic hydroxyl groups of the meso -diols are clearly differentiated by the stereochemistry at the C2 position of the glycosyl donor with excellent regioselectivities. In addition, the present method is successfully applied to the synthesis of core structures of phosphatidylinositolmannosides (PIMs) and glycosylphosphatidylinositol (GPI) anchors, and common β-mannoside structures of the LLBM-782 series of antibiotics. The desymmetrization of meso -diols is an attractive method for preparing chiral molecules bearing multiple stereogenic centers in one operation. Highly designed chiral catalysts possessing a nitrogen base on the chiral scaffold allow for the enantioselective functionalization [1] , [2] of meso -diols by desymmetrization reactions, such as acylation [3] , silylation [4] , [5] , and sulfonylation [6] (Fig. 1a ). In addition, other approaches, such as oxidation [7] , [8] , [9] , Heck reaction [10] , and lipase-catalyzed selective acylation [11] were also reported. However, the repertoire of enantio- or diastereoselective functionalization reactions of meso -diols is still limited. Therefore, to efficiently synthesize diversified valuable compounds from meso -diols, a new repertoire of desymmetric reactions has been in great demand. In this context, our interest was directed toward biosynthetic reactions that provide many biologically active natural products derived from meso -compounds. In nature, meso -compounds representing myo -inositol and 2-deoxystreptamine derivatives have been modified by enzymatic desymmetrization reactions, such as phosphorylation [12] and glycosylation [13] . With regard to phosphorylation, Miller et al. focused on the analogy of key intermediates between phosphorylation and acylation, and developed a pioneering highly enantioselective desymmetric phosphorylation of a myo -inositol derivative using chiral peptide catalysts discovered by screening a peptide library [14] , [15] . Recently, Fukase and Fujimoto et al. have reported another method for desymmetric phosphorylation of a myo -inositol derivative [16] . On the other hand, for glycosylation, despite the existence of many natural glycosides derived from meso -compounds, there is no method for the highly diastereoselective desymmetric glycosylation of meso -diols. Fig. 1: Enantio- or diastereoselective functionalizations of meso -diols. a Highly enantioselective functionalizations of meso -diols using highly designed chiral catalysts. b Synthetic strategy for myo -inositol glycoside from a meso -diol. c Boronic-acid-catalyzed desymmetric 1,2- cis -glycosylations of meso -diols. X leaving group, P protecting group, Ar aryl, Glc glucose, Gal galactose, Rha rhamnose, Man mannose, Fuc fucose. Full size image Highly diastereoselective desymmetric glycosylations of meso -diols can greatly increase the efficiency with which desymmetrized meso -compounds by glycosylations are prepared. As an example, the conventional synthetic strategy of myo -inositol glycoside is shown in Fig. 1b . In this strategy, myo -inositol glycosides were synthesized using a chiral auxiliary [17] , [18] . A meso -diol derived from myo -inositol was first functionalized using a chiral auxiliary, followed by stereoselective glycosylation of the desired diastereomer and finally, removal of the chiral auxiliary to give the desired myo -inositol glycoside. However, most desymmetrization methods of myo -inositol derivatives using a chiral auxiliary proceeded with low regioselectivity, providing a mixture with an undesired diastereomer. In addition, at least three steps were required to introduce the sugar moiety into the desired position in the myo -inositol derivatives. In another approach, optically pure myo -inositols were synthesized from d -glucose through Ferrier rearrangement [19] , however, a tedious multi-step operation was required. Thus, a highly diastereoselective desymmetric glycosylation of meso -diols would provide the desired myo -inositol glycosides in only one step. In the development of a desymmetric glycosylation of meso -diols, it is challenging to completely and simultaneously control both the α/β stereoselectivity of the anomeric center and the regioselectivity of the glycosylation site. Efficient stereoselective glycosylation methods have been developed for the α/β stereoselectivity [20] . However, there is no efficient desymmetric glycosylation method that can predict and concisely control the regioselectivity in the reaction with meso -diols. Although several cases of desymmetric α-mannosylations of meso -diols have been reported so far, the regioselectivities were low to moderate [21] , [22] . In addition, the regioselectivities of these glycosylations using other substrates are unpredictable because detailed reaction mechanisms and transition states during the glycosylations are still unclear. In this context, we focus on our organoboron-catalyzed 1,2- cis -glycosylations of 1,2-anhydro donors and mono-, di-, and poly-ol sugar acceptors [23] , [24] , [25] , [26] , [27] , [28] , [29] . The combination of a 1,2-anhydro donor and a boronic or borinic acid catalyst in the glycosylation gives excellent 1,2- cis -stereoselectivities. In addition, the S N i-type mechanism and the transition states are supported by mechanistic studies. Thus, we expect that the glycosylation of a 1,2-anhydro donor and a meso -diol using a boronic acid catalyst will give a 1,2- cis -glycoside with high stereoselectivity via the S N i-type mechanism, and the regioselectivity will be predictable by analyzing transition states with density functional theory (DFT) calculations. Herein, we report a highly diastereoselective desymmetric 1,2- cis -glycosylation of meso -diols found in myo -inositol 1,3,5-orthoesters using a boronic acid catalyst based on predictions of regioselectivity by DFT calculations (Fig. 1c ). The enantiotopic hydroxyl groups of the meso -diols are clearly differentiated by the stereochemistry at the C2 position of the 1,2-anhydro glycosyl donor with excellent regioselectivity. In addition, the present method is successfully applied to the synthesis of core structures of phosphatidylinositolmannosides (PIMs) and glycosylphosphatidylinositol (GPI) anchors, and common β-mannoside structure of the LLBM-782 series of antibiotics. Desymmetric glycosylations of myo -inositol derivatives To investigate our hypothesis, we first selected 1,2-anhydro- d -glucose 1 , 2- O -methyl- myo -inositol 1,3,5-orthoformate ( 2 ), and 4-nitrophenylboronic acid ( 3 ) as the glycosyl donor, meso -diol acceptor, and arylboronic acid, respectively, and investigated the transition states by DFT calculations (Fig. 2a , Supplementary Fig. 41 ). It was found that donor 1 could approach the boron atom from either the convex or concave face of boronic ester 4 , forming reasonable transition states in which the anomeric center of the donor is near the oxygen atom of the 4 position (TS-Glc-Convex) or 6 position (TS-Glc-Concave), respectively. The difference in activation energy was found to be 0.6 kcal mol −1 . These results indicated that the glycosylation at the 6 position via TS-Glc-Concave was favored over glycosylation at the 4 position via TS-Glc-Convex. The activation energy difference was caused by the ring strain in the envelope conformation of the dioxaborinane ring in TS-Glc-Convex, which was induced by steric hindrance between the aryl group of the boronic acid and the hydrogen atom at the 2 position of the meso -diol 2 . Therefore, we expected that the desymmetric glycosylation of 1,2-anhydro- d -glucose 7 and meso -diol 8 would proceed regioselectively to give the corresponding α(1,6)- d -glucoside 9 via the favored boat-type transition state similar to TS-Glc-Concave. Fig. 2: Desymmetric glycosylation using 1,2-anhydro-d-glucose. a Transition states calculated using B3LYP/6-31G* (single point energy: B3LYP/6-31+G**). b Desymmetric glycosylation of 7 and 8 . TS transition state, Me methyl, Bn benzyl, THF tetrahydrofuran, TBS tert -butyldimethylsilyl. Full size image To investigate our prediction, the desymmetric glycosylation of 7 and 8 using a catalytic amount of 3 was examined (Fig. 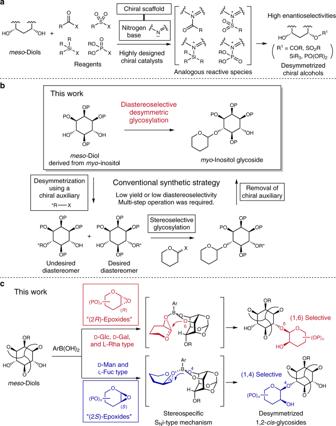Fig. 1: Enantio- or diastereoselective functionalizations ofmeso-diols. aHighly enantioselective functionalizations ofmeso-diols using highly designed chiral catalysts.bSynthetic strategy formyo-inositol glycoside from ameso-diol.cBoronic-acid-catalyzed desymmetric 1,2-cis-glycosylations ofmeso-diols. X leaving group, P protecting group, Ar aryl, Glc glucose, Gal galactose, Rha rhamnose, Man mannose, Fuc fucose. 2b , Supplementary Table 1 ). It was found that the glycosylation proceeded smoothly to provide α(1,6)- d -glucoside 9 in 96% yield with excellent regio- and stereoselectivities without forming any other regio- and stereoisomers 10 – 12 (Supplementary Figs. 2 , 3 , and 6 – 8 , Supplementary Tables 2 and 3 ). This observed regioselectivity was good agreement with the calculation result using the model compounds (Fig. 2a ). Since 1,2-anhydro donor 7 was the only chiral source in this glycosylation, the absolute configuration of stereogenic center(s) in the glycosyl donor was an origin of the excellent regioselectivity of this glycosylation. This result indicated that the chirality of the glycosyl donor was completely transferred to the meso -diol, leading to the clear differentiation of enantiotopic hydroxyl groups in meso -diols. The effect of protecting groups of the meso -diol using 13 – 15 was also examined (Fig. 3 ). The corresponding α(1,6)- d -glucosides 20 – 22 were obtained as single isomers in high yields (Supplementary Figs. 2 , 4 , and 9 – 12 , Supplementary Tables 4 – 9 ). In addition, even when triol 16 possessing a more reactive hydroxyl group at 2 position was used, α(1,6)- d -glucoside 23 was obtained with excellent diastereoselectivity (Supplementary Tables 10 and 11 ). This result indicated that the activation of 4,6-diol by the boronate ester formation was more important for the glycosylation than the innate reactivity of hydroxyl group. Next, the effect of protecting groups of the glycosyl donor using 17 – 19 (synthesis of 18 was described in Supplementary Fig. 1 ) was examined. In these cases, also, the desymmetric glycosylations proceeded effectively to give the corresponding α(1,6)- d -glucosides 24 – 26 with high regio- and 1,2- cis -stereoselectivities in high yields (Supplementary Figs. 2 , 5 , and 13 – 15 , Supplementary Tables 12 – 17 ). These results clearly indicated that the regioselectivity of the present glycosylations was not affected by the protecting groups. Fig. 3: Substrate scope of the protecting groups in the desymmetric glycosylation using 1,2-anhydro-d-glucose. Bz benzoyl, Ph phenyl, TBDPS tert-butyldiphenylsilyl. Full size image Construction of a prediction model We hypothesized that the regioselectivity was mainly affected by the C2 configuration of the glycosyl donor, and constructed a prediction model for the regioselectivities using (2 R )-epoxide donors, such as 1,2-anhydro- d -glucose, d -galactose, and l -rhamnose, and (2 S )-epoxide donors, such as 1,2-anhydro- d -mannose and l -fucose, as shown in Fig. 4a . 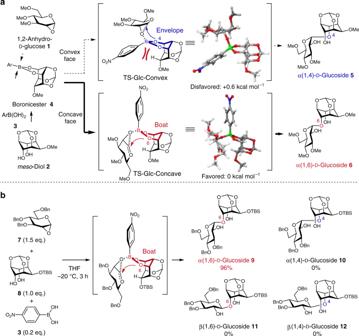Fig. 2: Desymmetric glycosylation using 1,2-anhydro-d-glucose. aTransition states calculated using B3LYP/6-31G* (single point energy: B3LYP/6-31+G**).bDesymmetric glycosylation of7and8. TS transition state, Me methyl, Bn benzyl, THF tetrahydrofuran, TBStert-butyldimethylsilyl. According to this model, it was expected that the glycosylations of (2 R )-epoxide donors would occur at the 6 position via boat-type transition states. On the other hand, in the cases of 1,2-anhydro donors possessing S configuration at the C2 position, the regioselectivity would be reversed and the glycosylations would occur at the 4 position. Fig. 4: Desymmetric glycosylation using several 1,2-anhydro donors. a Prediction model for regioselectivity. b Transition states calculated using B3LYP/6-31G* (single point energy: B3LYP/6-31+G**). The atoms colored gray, white, blue, red, and green in transition states represent C, H, N, O, and B, respectively. Full size image To validate this prediction model, we analyzed the boronic acid 3 catalyzed glycosylations of meso -diol 2 with several 1,2-anhydro glycosyl donors 27 – 29 by DFT calculations (Fig. 4b ). Using 1,2-anhydro- l -rhamnose 27 , two transition states were found in which the donor approached from the concave and convex faces of boronic ester 4 , i.e., TS-Rha-Concave which leads to β(1,6)- l -rhamnoside 30 and TS-Rha-Convex which leads to β(1,4)- l -rhamnoside 31 . As with 1,2-anhydro- d -glucose 1 , TS-Rha-Concave was favored over TS-Rha-Convex by 2.8 kcal mol −1 due to a similar ring strain of the envelope conformation, indicating that β-rhamnosylation using 1,2-anhydro- l -rhamnose would occur at the 6 position. Also, when 1,2-anhydro- d -mannose 28 and l -fucose 29 possessing the S configuration at the C2 position were used, the approach of these donors from the concave face to the boron atom was favored, similar to the (2 R )-epoxide donor, and the anomeric center of the glycosyl donor was positioned near the 4 position in the favored TSs (TS-Man-Concave and TS-Fuc-Concave) as expected, indicating that β-mannosylation and α-fucosylation would proceed regioselectively at the 4 position. These predictions of regioselectivities by DFT calculations were in good agreement with the prediction model, suggesting that the regioselectivity of the present glycosylation reaction was attributed to the stereochemistry at C2 of the glycosyl donor. In fact, we investigated the glycosylations of several 1,2-anhydro donors and meso -diol 8 (Fig. 5 ). Using 1,2-anhydro- d -galactose 36 , similarly to 1,2-anhydro- d -glucose 7 , α(1,6)- d -galactoside 40 was obtained in high yield with high regio- and stereoselectivities (Supplementary Figs. 16 – 18 , Supplementary Tables 18 and 19 ). The use of 1,2-anhydro- l -rhamnose 37 gave β(1,6)- l -rhamnoside 42 as a single isomer as expected (Supplementary Figs. 19 – 21 , Supplementary Tables 20 and 21 ). Also, when 1,2-anhydro- d -mannose 38 was used, β-mannosylation occurred at the 4 position in 8 according to our prediction model, and β(1,4)- d -mannoside 43 was obtained with complete regio- and stereoselectivities (Supplementary Figs. 22 – 24 , Supplementary Tables 22 and 23 ). Similarly, the glycosylation using 1,2-anhydro- l -fucose 39 proceeded regioselectively to give α(1,4)- l -fucoside 44 in good yield (Supplementary Figs. 25 – 27 , Supplementary Tables 24 , 25 ). All of these obtained experimental regioselectivities were in good agreement with our prediction model, clearly demonstrating that the regioselectivity of the present desymmetric glycosylation can be easily predicted. Fig. 5: Substrate scope of the glycosyl donors in the desymmetric glycosylation of 8 . In all cases, the formation of 1.2- trans glycoside was not observed. Full size image Application to acyclic meso -diols Next, as a preliminary attempt, we examined the desymmetric glycosylations of acyclic meso -diols, which possess high conformational flexibility, to show the possibility of the present glycosylation method (Fig. 6 ). The results showed that when acyclic meso -diols 45 and 48 were used, the glycosylations proceeded smoothly to provide the corresponding 1,2- cis -glycosides in high yields with moderate and excellent regioselectivities, respectively, and excellent 1,2- cis -α-stereoselectivities (Supplementary Figs. 30 – 37 , Supplementary Tables 28 – 31 ). Although the rationale of regioselectivities was still unclear, these results showed the possibility that this glycosylation method could be applicable to acyclic meso -diols. Further investigations using several acyclic meso -diols is now in progress in our laboratory. Fig. 6: Desymmetric glycosylation using acyclic meso -diols. In both cases, the formation of 1.2- trans glycoside was not observed. Full size image Synthesis of core structures of PIMs and GPI anchors Overall, we developed the highly diastereoselective desymmetric 1,2- cis -glycosylation, which can be able to synthesize various 1,2- cis -glycosides. Next, we focused on the representative myo -inositol glycosides, PIMs and GPI anchors (Fig. 7a ). Although several synthetic strategies have been developed for PIMs [19] , [21] , [30] , [31] , [32] , [33] , [34] , [35] , [36] , [37] , [38] , [39] and GPI anchors [17] , [18] , [40] , [41] , [42] , [43] , [44] , [45] , [46] , which possess α-mannose and α-glucosamine at 6 position of myo -inositol, respectively, there are few efficient methods for highly regio- and stereoselective introduction of these sugars. Therefore, the efficient synthesis of core structures of PIMs and GPI anchors using the present glycosylation as a key step was examined (Fig. 7b , Supplementary Figs. 38 and 39 ). Initially, selective triflation of 9 and displacement using CsOAc, followed by deprotection of TBS group, afforded α(1,6)- d -mannoside 50 . Mannosylation at the 2 position in inositol moiety provided core structure 52 of PIMs. In addition, protection of 9 using benzoyl and methoxymethyl (MOM) groups, followed by deprotection of benzoyl group, gave 53 . Finally, oxidation and oximation, followed by reduction, afforded core structure 54 of GPI anchors. These results indicated that the present glycosylation method could lead to synthesize PIMs and GPI anchors effectively. Fig. 7: Synthetic scheme of core structures of PIMs and GPI anchors. a Chemical structures of PIMs and GPI anchors. b Synthesis of core structures 52 and 54 using the present glycosylation method. Tf trifluoromethanesulfonyl, Ac acetyl, TBAF tetra- n -butylammonium fluoride, Et ethyl, MS molecular sieve, MOM methoxymethyl, DIPEA N , N -diisopropylethylamine, BRSM based on recovered starting material. Full size image Synthesis of common structure of the LLBM-782 series Finally, we applied the glycosylation method to the synthesis and structural determination of a common mannosyl inositol structure of the LLBM-782 series of antibiotics [47] , [48] , [49] . The β configuration of the anomeric center was supported by the 1 J CH value of LLBM-782α 2 (163.9 Hz) [48] , [49] . However, in general, it is difficult to judge the anomeric configuration to be α or β using this ambiguous 1 J CH value [50] , [51] . Therefore, in order to determine the anomeric configuration of the LLBM-782 series, we planned to synthesize common β-mannoside structure 55 β of the LLBM-782 series using the present glycosylation method, and compare it to mannoside 55 , which was provided by base hydrolysis of LLBM-782α 1 [47] as shown in Fig. 8a . Fig. 8: Synthetic scheme of mannoside 55 β. a Chemical structures of LLBM-782 series and mannoside 55 produced by base hydrolysis of LLBM-782α 1 . b Synthesis of mannoside 55 β using the present glycosylation method. PMB p -methoxybenzyl, DMF dimethylformamide. Full size image The synthetic scheme of 55 β is shown in Fig. 8b (Supplementary Fig. 40 ). Desymmetric glycosylation of 1,2-anhydro- d -mannose 56 and meso -diol 8 proceeded efficiently to provide β(1,4)- d -mannoside 57 in high yield as a single isomer (Supplementary Figs. 28 and 29 , Supplementary Tables 26 and 27 ). The anomeric configuration of 57 was confirmed by 1 J CH of the anomeric center (159 Hz) and nOe experiments. Deprotection of the orthoformate and TBS groups, followed by benzylation, gave 58 in good yield. Deprotection of the PMB group and oxidation, followed by oximation, afforded oxime 59 . Acetylation, reduction, and carbamoylation gave protected urea 60 . Deprotection of the benzyl groups in 60 furnished structurally defined β-mannoside 55 β. 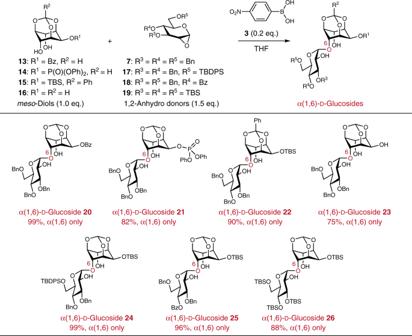Fig. 3: Substrate scope of the protecting groups in the desymmetric glycosylation using 1,2-anhydro-d-glucose. Bz benzoyl, Ph phenyl, TBDPS tert-butyldiphenylsilyl. The 13 C-NMR spectrum of the analytical sample of 55 β was identical to the reported data for mannoside 55 [47] (Supplementary Table 32 ), indicating that the anomeric configuration of LLBM-782 series is β. In conclusion, we developed a method for the diastereoselective desymmetric 1,2- cis -glycosylation of meso -diols by using a combination of 1,2-anhydro donors and boronic acid catalyst. High regioselectivities of the glycosylations were predicted by DFT calculations, and those were in good agreement with our experimental regioselectivities. The difference in regioselectivities using several 1,2-anhydro donors was attributed to the stereochemistry at the C2 position of the glycosyl donor. The present glycosylation method was applied to the synthesis of core structures of PIMs and GPI anchors, and common β-mannoside structure 55 β of the LL-BM782 series of antibiotics. Further applications of this glycosylation method to the synthesis of various glycosides possessing meso -structures are now in progress in our laboratory. Materials For 1 H- and 13 C-NMR spectra of compounds in this study, see Supplementary Information (Supplementary Figs. 42 – 125 ). 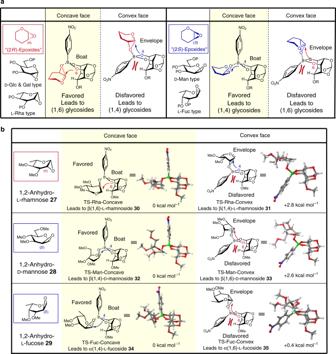Fig. 4: Desymmetric glycosylation using several 1,2-anhydro donors. aPrediction model for regioselectivity.bTransition states calculated using B3LYP/6-31G* (single point energy: B3LYP/6-31+G**). The atoms colored gray, white, blue, red, and green in transition states represent C, H, N, O, and B, respectively. For the detailed synthetic procedures and methods of DFT calculations, see Supplementary Information. For the data of DFT calculations, see Supplementary Dataset 1. 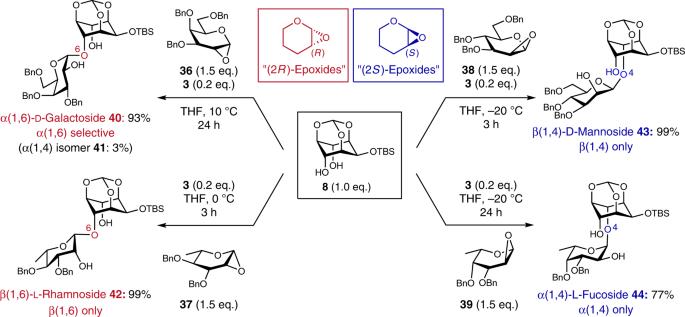Fig. 5: Substrate scope of the glycosyl donors in the desymmetric glycosylation of8. In all cases, the formation of 1.2-transglycoside was not observed. General procedure for desymmetric glycosylation To a solution of meso -diol (0.02–0.05 mmol, 1.0 equiv.) and p -nitrophenylboronic acid ( 3 ) (4–10 μmol, 0.2 equiv.) in dry THF (0.2 M to meso -diol) was added a solution of 1,2-anhydro donor (0.03–0.15 mmol, 1.5–3.0 equiv.) in dry THF (0.2 M to 1,2-anhydro donor) at the temperature indicated under Ar atmosphere. After the reaction mixture was stirred for 3 h, the reaction was quenched by addition of 0.05 M NaBO 3 aq. (8.8–22 μmol, 0.44 equiv.). To the resultant mixture was added sat. NH 4 Cl aq. (2 mL). The aqueous layer was extracted with EtOAc (3 mL × 3), and then the combined extracts were washed with brine (5 mL), dried over anhydrous Na 2 SO 4 , and concentrated in vacuo . 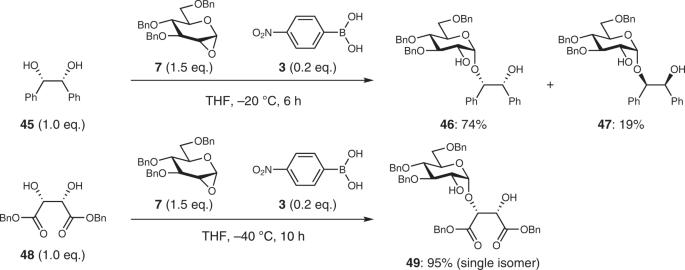Fig. 6: Desymmetric glycosylation using acyclicmeso-diols. In both cases, the formation of 1.2-transglycoside was not observed. 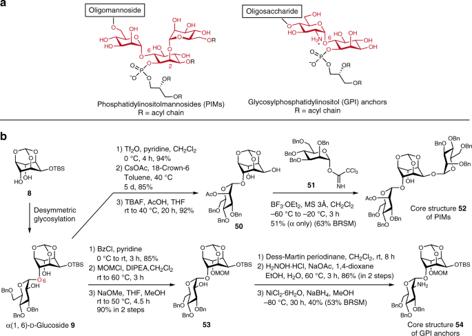Fig. 7: Synthetic scheme of core structures of PIMs and GPI anchors. aChemical structures of PIMs and GPI anchors.bSynthesis of core structures52and54using the present glycosylation method. Tf trifluoromethanesulfonyl, Ac acetyl, TBAF tetra-n-butylammonium fluoride, Et ethyl, MS molecular sieve, MOM methoxymethyl, DIPEAN,N-diisopropylethylamine, BRSM based on recovered starting material. 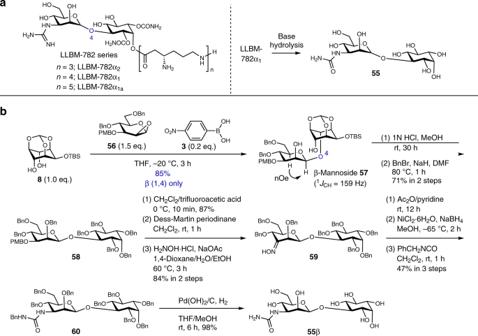Fig. 8: Synthetic scheme of mannoside55β. aChemical structures of LLBM-782 series and mannoside55produced by base hydrolysis of LLBM-782α1.bSynthesis of mannoside55β using the present glycosylation method. PMBp-methoxybenzyl, DMF dimethylformamide. The crude material was purified by column chromatography on SiO 2 .